Physiological sodium concentrations enhance the iodide affinity of the Na+/I−symporter The Na + /I − symporter (NIS) mediates active I − transport—the first step in thyroid hormonogenesis—with a 2Na + :1I − stoichiometry. NIS-mediated 131 I − treatment of thyroid cancer post-thyroidectomy is the most effective targeted internal radiation cancer treatment available. Here to uncover mechanistic information on NIS, we use statistical thermodynamics to obtain K d s and estimate the relative populations of the different NIS species during Na + /anion binding and transport. We show that, although the affinity of NIS for I − is low ( K d =224 μM), it increases when Na + is bound ( K d =22.4 μM). However, this K d is still much higher than the submicromolar physiological I − concentration. To overcome this, NIS takes advantage of the extracellular Na + concentration and the pronounced increase in its own affinity for I − and for the second Na + elicited by binding of the first. Thus, at physiological Na + concentrations, ~79% of NIS molecules are occupied by two Na + ions and ready to bind and transport I − . The thyroid hormones—T 3 and T 4 —are required for the development and maturation of the central nervous system, skeletal muscle, and lungs and for the regulation of intermediate metabolism in all cells throughout life [1] . Iodine, a scarce element, is an essential constituent of these hormones. The Na + /I − symporter (NIS) is the key plasma membrane protein that mediates active I − uptake in the thyroid and other tissues, such as lactating breast, salivary glands, stomach and intestine [2] , [3] , [4] . NIS is also at the centre of the highly effective thyroid cancer treatment involving administration of radioiodide after thyroidectomy, a strategy that has been used for over 65 years [5] , [6] , [7] , [8] . Despite the obvious pathophysiological significance of NIS, it was not until 1996 that its cDNA was cloned [9] , making it possible to use gene transfer protocols in pre-clinical and clinical studies to extend NIS-mediated radioiodide treatment to extrathyroidal cancers [10] , [11] . Active accumulation of I − by NIS is electrogenic, with a stoichiometry of two Na + ions per transported I − (2:1), and uses as its driving forces the Na + gradient generated by the Na + /K + ATPase and the electrical potential across the plasma membrane [9] , [12] . The total driving force provided by the downhill movement of Na + ions under typical conditions ([Na + ] extracellular =140 mM; [Na + ] intracellular =14 mM; membrane potential nearly −60 mV; temperature=37 °C) is ~4.3 kcal mol −1 . Under these conditions, given the cost of transporting I − against its concentration gradient and against the membrane potential, the maximum attainable I − gradient {[I − ] i /[I − ] e } max is ≤1,000. However, the maximum amount of I − that can be accumulated does not depend only on the driving force: all the individual steps in the process (binding of extracellular ions, translocation of the ions across the membrane and release of the ions into the cytoplasm) have to be thermodynamically feasible and kinetically competent. Significant advances have been made in the molecular characterization of NIS—for example, in elucidating its transcriptional and posttranscriptional regulation and in uncovering its structure–function relations [13] , [14] , [15] , [16] , [17] , [18] , [19] . NIS has been demonstrated to transport both perrhenate (ReO 4 − ) and the environmental pollutant perchlorate (ClO 4 − ) electroneutrally, indicating that it transports different substrates with different stoichiometries [20] . However, little is known about how its substrates are bound and released—a fundamental mechanistic question. To address this gap in our knowledge, we devised a new approach. We analysed kinetic data using statistical thermodynamics, and determined the affinity of the symporter for the transported ions as well as the relative populations of the different NIS species present during the transport cycle. Whereas a similar approach has been used to study repressor regulation using binding data [21] , [22] , [23] , [24] and to analyse protein-folding data [25] , [26] , [27] , the results presented here show that this approach can also be employed to obtain mechanistic information on transporters and channels and could complement energy landscape studies, such as those that have been carried out on ion-translocating ATPases [28] . We show that the low affinity of NIS for I − ( K d =224 μM) increases ( K d =22.4 μM) when Na + is bound, and that at physiological extracellular Na + concentrations, as many as ~79% of NIS molecules are occupied by two Na + ions and thus poised to bind and transport I − . The statistical thermodynamics approach presented here promises to be applicable to other transporters and channels, including those of medical importance. Remarkably, this approach makes it possible to obtain quantitative mechanistic information about these proteins in their native environment—whole cells—without the need for membrane protein purification. Transport by NIS Initial rates of transport were assessed for WT NIS in the intestinal epithelial cell line IEC-6 (refs 2 , 29 ) using either 125 I − or 186 ReO 4 − . IEC-6 cells were used because, as we have reported previously, they express NIS at higher levels than FRTL-5 cells, the rat thyroid cells from which NIS was originally cloned [9] . In addition, NIS in IEC-6 cells has the same apparent affinity for its substrates as NIS in FRTL-5 cells [2] , [29] . I − transport was measured in five experiments, three varying [Na + ] at three or four [I − ]s and two varying [I − ] at five [Na + ]s (one example of each is shown in Supplementary Fig. 1a ). Initial rates of ReO 4 − transport were measured in four different experiments, two varying [Na + ] at four different [ReO 4 − ]s, and two varying [ReO 4 − ] at four different [Na + ]s (one example of each is shown in Supplementary Fig. 2a ). The individual curves were fitted by least squares to the Michaelis–Menten equation. In all cases, the K M for the ion being varied depends strongly on the concentration of the other ion, indicating that binding of either ion to empty NIS increases the protein’s affinity for the other ion. Interpretation of these observations requires a theoretical context beyond the Michaelis–Menten formulation. Theoretical background Transporters such as NIS are expected to exist in at least two conformations [30] , [31] , [32] , [33] : one in which they are open to the extracellular milieu and bind the ions to be transported, and one in which they are open to the cytoplasm and release the ions. Since NIS carries out coupled transport involving three ions (2 Na + and 1 I − ), it must have three binding sites—one for each of the transported ions. In principle, each site may be occupied at any time, by itself or in combination with occupation of the other sites. The eight different molecular species of the outwardly open conformation (no ions bound, one Na + site occupied, the other Na + site occupied, and so on) and the relations between them are shown in Fig. 1 , where each of the eight states is a corner of the cube and each edge represents a reaction involving binding an additional ion. These states represent not only the addition of the ion but also the conformational changes that result from binding the ion. (In principle, these conformations exist even in the absence of the ions [34] , [35] , but in the present analysis they are considered of too-low occupancy to influence the results). 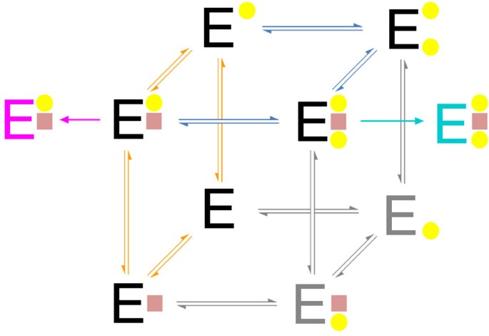Figure 1: States contributing to I−and ReO4−transport. E represents NIS. The upper yellow circle is the bound Na+to site NaA; the lower one, bound NaB. The mauve square is bound I−or ReO4−. The blue, orange and grey arrows represent ion binding. The cyan arrow represents the switch from the outwardly to the inwardly facing conformation for I−transport; the magenta arrow, the same switch for ReO4−transport. The states represented in grey were shown not to be significantly occupied during the transport cycle. The Na+sites designated A and B in the text refer only to the order of binding and do not necessarily correspond to the crystallographically identified ‘site 1’ and ‘site 2’ of LeuT30. Figure 1: States contributing to I − and ReO 4 − transport. E represents NIS. The upper yellow circle is the bound Na + to site NaA; the lower one, bound NaB. The mauve square is bound I − or ReO 4 − . The blue, orange and grey arrows represent ion binding. The cyan arrow represents the switch from the outwardly to the inwardly facing conformation for I − transport; the magenta arrow, the same switch for ReO 4 − transport. The states represented in grey were shown not to be significantly occupied during the transport cycle. The Na + sites designated A and B in the text refer only to the order of binding and do not necessarily correspond to the crystallographically identified ‘site 1’ and ‘site 2’ of LeuT [30] . Full size image Assuming that only the triply occupied NIS can switch to the inwardly open conformation, and that this conformational change is slow or much less frequent than the binding and unbinding of ions, all eight species can be considered to be in equilibrium. This assumption can be relaxed to include the case in which other states can transition to the inwardly open conformation, but this happens infrequently. These transitions may be responsible for the Na + leak observed in electrophysiological experiments [12] . Twelve equilibrium constants (one per edge) define the equilibrium between the eight species. However, the four constants on each face of the cube are not independent: going from one corner of any face to the opposite corner of the same face produces the same species independently of the path taken; in other words, the two possible paths are thermodynamically equivalent. Since there are six faces providing an equal number of equations relating equilibrium constants, only six independent constants are necessary to fully describe the system. We chose as our constants the association constant of each of the three ions for the empty NIS molecule ( , where is the standard molar free energy of binding of ion X to the empty transporter) and φ x,y ( ) is the enhancement in affinity for ion X that results from having ion Y bound (Δ g x,y reflects the increase in the free energy of the interaction; see Supplementary Table 1 ). The fraction of NIS molecules in each of these states is proportional to its statistical thermodynamics weight exp( −ΔG i / RT ), where ΔG i is the free energy of state i with respect to the empty NIS molecule, which is defined as the ground state. ΔG i is given by where is the standard molar Gibbs free energy of binding of the ions to the empty transporter and {[ X x ]} represents the product of the concentrations (activities) of the ions X that are bound to the protein in state i (see Supplementary Table 1 ). In turn, is expanded as the intrinsic standard molar free energy of binding of each ion to the empty transporter, , plus the free energy of interaction between pairs of bound ions, Δ g x,y . The eight states and their statistical weights are given in Supplementary Table 1 , where the statistical weights ξ i are expanded as In this expression, { K a,x } is the product of the association constants of all the ions in species i to the empty transporter, { φ x,y } is the product of the enhancement factors of binding ions x and y to the same molecule and {[ X x ]} is the product of the concentrations of the free ions in state i . The partition function Q is obtained as the sum of all statistical weights ( Q =∑ ξ i ). These considerations lead to equation (3) for I − transport (see Supplementary Table 1 for the definition of states and their statistical weights). with The fraction of protein molecules in state i can be calculated by dividing the statistical weight of state i by the partition function ( f i =ξ i / Q ). NIS transports the anion perrhenate (ReO 4 − ) with a 1:1 stoichiometry: one ReO 4 − is transported using only one Na + (ref. 20 ), and therefore, its kinetics depend on [Na + ] and not on [Na + ] 2 . The processes leading to ReO 4 − transport correspond to the orange arrows on the leftmost face of the cube in Fig. 1 . The species with two bound Na + ions may also have a significant occupancy even if it does not contribute to ReO 4 − transport. Assuming that only the doubly occupied species can transport ReO 4 − and that the transition from outwardly to inwardly open is slow compared to ion binding and unbinding, the rate of transport is proportional to v max times the fraction of doubly occupied NIS molecules (Na + and ReO 4 − bound). Under these conditions, all four species are at equilibrium, and therefore, the proportion of the different species can also be determined using a statistical thermodynamics approach. Using the same formulation as for I − , the rate of ReO 4 − transport by NIS is given by with The constants can be obtained by non-linear least-squares fitting of initial velocities of transport at different concentrations of Na + and ReO 4 − . Importantly, these constants will include a value for K a,NaA , the apparent affinity of Na + for free NIS. This value is independent of the anion being transported and can therefore be used directly in the equation for I − transport. ReO 4 − transport Initial rates of ReO 4 − transport were measured in the intestinal epithelial cell line IEC-6 (refs 2 , 29 ) in four different experiments, two varying [Na + ] at four different [ReO 4 − ]s and two varying [ReO 4 − ] at four different [Na + ]s (see one example of each in Supplementary Fig. 2a ). Attempts to find values for the six parameters in the equation— K a , NaA , K a , NaB , K a , ReO4 , φ Na,ReO4 , φ NaA,NaB and v max —by non-linear least-squares fit of the normalized initial rates of 232 experimental points were unsuccessful until the terms that contain K a , NaB were removed and the data were analysed using equation (5), which includes a single Na + site. The values obtained for the four parameters are shown in Table 1 . The data show that the empty transporter has a low affinity for both ions ( K d s: 137 mM for Na + and 29.8 μM for ReO 4 − ). These constants are real K d s because they reflect binding to the empty NIS molecule before the Michaelis–Menten complex is formed by binding the other ion. The affinity of NIS for each ion increases by a factor of 5.3 when the other ion is bound, resulting in K d s of 26 mM for Na + when ReO 4 − is already bound and 5.7 μM for ReO 4 − when Na + is already bound ( Table 1 ). These last constants are technically similar to K M s but they are equivalent to K d s as long as the assumption that the conformational transition from outwardly to inwardly open is much slower than ion unbinding is met. These K d s would be observed for each ion at saturating concentrations of the other ion. Table 1 Dissociation constants for I − and ReO 4 − transport by NIS and G93T NIS. Full size table It is surprising that occupancy of NaB is not compatible with the ReO 4 − transport data. The simplest explanation for this effect is that ReO 4 − binds to a high-affinity site in NIS (the ReO 4 HA site, for High Affinity) that is not involved in transport but prevents binding of Na + to the NaB site. This interpretation is further supported by the data on the NIS G93T mutant (see below). The rate of transport as a function of [Na + ] and [ReO 4 − ] can be calculated by substituting the fitted parameters into equation (5); ( Fig. 2a ). Furthermore, the same parameters can be used to calculate the fraction of each of the other three species—E, E Na and E ReO4 —by replacing the numerator in equation (5) with its statistical weight (1.0, K a,Na [ Na + ] and K a,ReO 4 [ ReO 4 − ]). The results show that, even at high concentrations of either ion, the fraction of empty NIS molecules remains high ( Fig. 2b ), but this fraction approaches zero when both ions are present. For either ion, the fraction of species with only that ion bound decreases rapidly when the concentration of the other ion is increased ( Fig. 2c,d ). Also, at physiological extracellular [Na + ] (140 mM; black circles in Fig. 2a ) the rate of transport increases very rapidly with increasing [ReO 4 − ]. 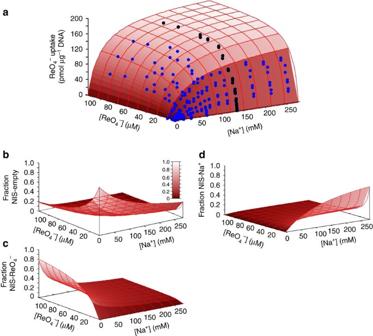Figure 2: Statistical thermodynamics analysis of ReO4−transport by NIS. (a) Kinetic data for ReO4−transport expressed in pmol μg−1DNA. Blue circles represent the experimental rates. Black circles correspond to experimental values measured at 140 mM Na+, the physiological [Na+]. The surface represents the rate of transport calculated asvmaxtimes the fraction of molecules with Na+and ReO4−bound. (b) Fraction of empty NIS molecules. (c) Fraction of NIS molecules with ReO4−bound. (d) Fraction of NIS molecules with one Na+bound. Figure 2: Statistical thermodynamics analysis of ReO 4 − transport by NIS. ( a ) Kinetic data for ReO 4 − transport expressed in pmol μg −1 DNA. Blue circles represent the experimental rates. Black circles correspond to experimental values measured at 140 mM Na + , the physiological [Na + ]. The surface represents the rate of transport calculated as v max times the fraction of molecules with Na + and ReO 4 − bound. ( b ) Fraction of empty NIS molecules. ( c ) Fraction of NIS molecules with ReO 4 − bound. ( d ) Fraction of NIS molecules with one Na + bound. Full size image Iodide transport Initial rates of I − transport were measured in five experiments, three varying [Na + ] at three or four [I − ]s, and two varying [I − ] at five [Na + ]s (total 254 experimental points; see one example of each in Supplementary Fig. 1a ). Analysis of the initial rates of I − transport using equation (3) were carried out using 137 mM—the dissociation constant obtained by fitting the ReO 4 − data to equation (5)—as the K d , NaA . The non-linear least-squares fit was unstable until the species with the second (NaB) but not the first Na + (NaA) bound were neglected. The final parameters ( Table 1 ) show that when the first Na + site (NaA) is occupied, the affinity of the second Na + site (NaB) is increased significantly, exceeding even the affinity of the empty transporter for the first Na + (NaA). This affinity is similar to that of the first site (NaA) when I − is bound to NIS ( K d,NaA / φ NaA,I =17.6 mM). Similarly, empty NIS binds I − with low affinity ( K d =224 μM), but this affinity is greatly increased (10-fold) when Na + is bound to the first site (NaA). Tests designed to probe whether binding of the second Na + (NaB) further increases NIS’s affinity for I − showed no statistically significant increase in affinity. With these parameters, the initial rates of I − transport can be calculated as a function of all [Na + ]s and [I − ]s ( Fig. 3a ). As expected [9] , [12] , [14] , the dependence on [Na + ] is sigmoidal, while the dependence on [I − ] is hyperbolic ( Fig. 3a ). As in the case of ReO 4 − , the same parameters can be used to estimate the fractional occupancy of all species as a function of the concentration of the transported ions ( Fig. 3b–g ). At high [Na + ] and [I − ], the triply occupied species (2 Na + and 1 I − ) is essentially the only one present ( Fig. 3g ). Also, even at [I − ]=0, the species with a single Na + ion bound becomes unpopulated at high [Na + ] ( Fig. 3d ) because the affinity of NIS for the second Na + ion becomes higher when the first is bound, increasing the population of the species with two Na + ions ( Fig. 3f ). Since the affinity of NIS for I − is low in the absence of Na + , at [Na + ]=0 there is a substantial fraction of empty NIS even at high [I − ] ( Fig. 3b ). The increase in Na + affinity brought about by binding of I − is reflected in the rapid disappearance of empty NIS molecules when the [Na + ] increases even slightly ( Fig. 3b ). 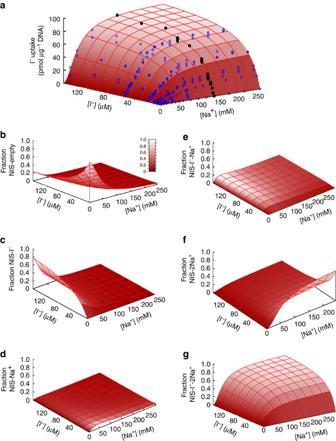Figure 3: Statistical thermodynamics analysis of I−transport by NIS. (a) Kinetic data for I−transport expressed in pmol μg−1DNA. Blue circles represent the experimental rates. Black circles correspond to experimental values measured at 140 mM Na+, the physiological [Na+]. The surface represents the rate of transport calculated asvmaxtimes the fraction of molecules with two Na+ions and one I−. (b) Fraction of empty NIS molecules. (c) Fraction of NIS molecules with I−bound. (d) Fraction of NIS molecules with one Na+bound. (e) Fraction of NIS molecules with two Na+ions bound. (f) Fraction of NIS molecules with I−and one Na+bound. (g) Fraction of NIS molecules with I−and two Na+bound (same asFig. 3abut normalized to 1.0 to reflect the fraction of EI−2Namolecules). Figure 3: Statistical thermodynamics analysis of I − transport by NIS. ( a ) Kinetic data for I − transport expressed in pmol μg −1 DNA. Blue circles represent the experimental rates. Black circles correspond to experimental values measured at 140 mM Na + , the physiological [Na + ]. The surface represents the rate of transport calculated as v max times the fraction of molecules with two Na + ions and one I − . ( b ) Fraction of empty NIS molecules. ( c ) Fraction of NIS molecules with I − bound. ( d ) Fraction of NIS molecules with one Na + bound. ( e ) Fraction of NIS molecules with two Na + ions bound. ( f ) Fraction of NIS molecules with I − and one Na + bound. ( g ) Fraction of NIS molecules with I − and two Na + bound (same as Fig. 3a but normalized to 1.0 to reflect the fraction of E I−2Na molecules). Full size image ReO 4 − transport by G93T NIS To further test the approach put forth here, we measured and analysed ReO 4 − transport by a NIS mutant (G93T NIS) with a remarkable property—namely, that it transports ReO 4 − electrogenically, with a 2 Na + : 1 ReO 4 − stoichiometry, which stands in contrast to the 1:1 stoichiometry of WT NIS [13] . Our analysis reveals that the mutation allows G93T NIS to use 2 Na + ions to transport ReO 4 − . The most straightforward explanation for this change in stoichiometry is that the mutation causes the loss of binding of ReO 4 − to the high-affinity ReO 4 HA site proposed above. The binding of ReO 4 − to this site is the reason Na + does not bind to the NaB site even in the presence of very low concentrations of ReO 4 − . By disrupting the binding of ReO 4 − to the ReO 4 HA site, the mutation allows binding of Na + to the NaB site and its participation in ReO 4 − transport. In addition, under all conditions—empty NIS, NIS with one Na + bound, NIS with one ReO 4 − bound, and so on—the affinity of the mutant for both ions is severely reduced ( Table 1 ). Nevertheless, ReO 4 − transport by the G93T NIS mutant mimics I − transport by WT NIS in that the initial rates of ReO 4 − transport by the mutant as a function of [Na + ] ( Fig. 4a ) show the expected sigmoidal [Na + ] dependence that indicates electrogenic transport, albeit shifted to much higher [Na + ]s. The calculated fractions of the different species ( Fig. 4b–g ) also show the tendencies that correspond to reduced affinities. 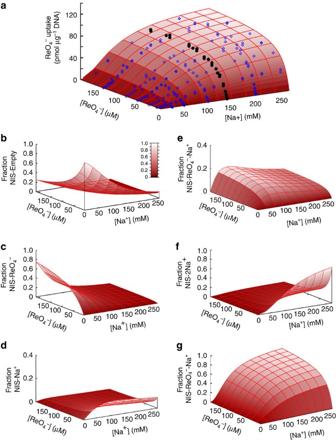Figure 4: Statistical thermodynamics analysis of ReO4−transport by G93T NIS. (a) Initial rates of ReO4−transport expressed in pmol μg−1DNA. Blue circles represent the experimental data. Black circles correspond to experimental values measured at 140 mM Na+, the physiological [Na+]. The surface represents the rate of transport calculated asvmaxtimes the fraction of molecules with two Na+ions and one I−. (b) Fraction of empty NIS molecules. (c) Fraction of NIS molecules with ReO4−bound. (d) Fraction of NIS molecules with one Na+bound. (e) Fraction of NIS molecules with two Na+ions bound. (f) Fraction of NIS molecules with ReO4−and one Na+bound. (g) Fraction of NIS molecules with ReO4−and two Na+ions bound (same asFig. 3abut normalized to 1.0 to reflect the fraction of EI−2Namolecules). Figure 4: Statistical thermodynamics analysis of ReO 4 − transport by G93T NIS. ( a ) Initial rates of ReO 4 − transport expressed in pmol μg −1 DNA. Blue circles represent the experimental data. Black circles correspond to experimental values measured at 140 mM Na + , the physiological [Na + ]. The surface represents the rate of transport calculated as v max times the fraction of molecules with two Na + ions and one I − . ( b ) Fraction of empty NIS molecules. ( c ) Fraction of NIS molecules with ReO 4 − bound. ( d ) Fraction of NIS molecules with one Na + bound. ( e ) Fraction of NIS molecules with two Na + ions bound. ( f ) Fraction of NIS molecules with ReO 4 − and one Na + bound. ( g ) Fraction of NIS molecules with ReO 4 − and two Na + ions bound (same as Fig. 3a but normalized to 1.0 to reflect the fraction of E I−2Na molecules). Full size image The dissociation constants for Na + binding by another eukaryotic Na + driven transporter, the human glucose transporter hSGLT1, have been determined using electrophysiological methods [36] . Interestingly, the affinity for Na + of this transporter is very similar to that determined for NIS using our statistical thermodynamics approach ( K d =51 mM for NIS, Table 1 ; K d =20 mM for hSGLT1, (ref. 36 )). Fractional occupancies have been determined for another Na + -driven eukaryotic transporter, the NaPi-IIa/b phosphate transporter, using electrophysiological experiments [37] . The affinities we determined ( Table 1 ) can be converted into standard molar free energies using the relation Δ G o =− RT ln K . The free energies of association of Na + and I − to NIS were combined to yield the free energies of the individual species as a function of the transport reaction coordinate ( Fig. 5 ). The data show that the molecular species become more stable as their ion occupancy increases. Molecular dynamics calculations with other transporters also suggest that Na + binding stabilizes the outwardly facing conformation [31] , [38] , [39] , [40] , [41] . 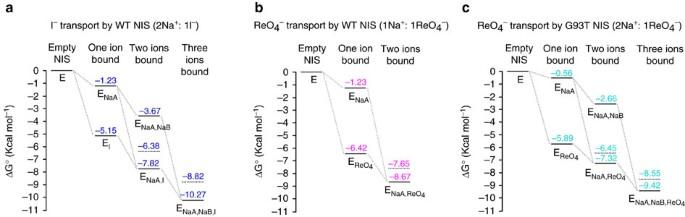Figure 5: Standard molar free energies of the species along the NIS transport reaction coordinate. The values of the standard molar free energies are shown along the vertical axis. The continuous lines show the standard molar free energy of each state (ΔGo) and the dotted lines show the value of ΔGoof the same state before the stabilization free energy Δgis added. (a) WT NIS transport of I−. (b) WT NIS transport of ReO4−. (c) G93T NIS transport of ReO4−. Figure 5: Standard molar free energies of the species along the NIS transport reaction coordinate. The values of the standard molar free energies are shown along the vertical axis. The continuous lines show the standard molar free energy of each state (Δ G o ) and the dotted lines show the value of Δ G o of the same state before the stabilization free energy Δ g is added. ( a ) WT NIS transport of I − . ( b ) WT NIS transport of ReO 4 − . ( c ) G93T NIS transport of ReO 4 − . Full size image The values in Table 1 can be used to calculate the intrinsic stabilities (as reflected in the Δ G o s; see Supplementary Table 1 ) of the different NIS molecular species present during transport in the three cases studied ( Fig. 5 ). In all three cases, binding of the first ion results in a more stable species, and binding of additional ions increases stability further. The details of how these effects favour anion transport are different in the three cases. WT NIS is modestly stabilized by binding of I − or one Na + (that is, the affinity of empty NIS for either ion is low). NIS compensates for this liability by increasing the stability of the species with I − and Na + bound by the amount Δg NaA,I , beyond the straightforward sum of the Δ G o s of the individual species ( Fig. 5a and Supplementary Table 1 ). A further increase in stability is brought about by binding of Na + to NaB. In ReO 4 − transport ( Fig. 5b ), the higher stability of the NIS species with ReO 4 − bound and the increment in affinity when Na + and ReO 4 − are both bound partially compensate for the non-binding of NaB. G93T NIS has a very low affinity for Na + compared with WT NIS; as a result, the G93T NIS species with one Na + bound has a lower stability than WT ( Fig. 5c ). This is partially compensated for by the fact that binding of ReO 4 − to G93T NIS stabilizes the NIS molecule more than binding of I − to WT NIS does (that is, the affinity of binding of ReO 4 − to G93T is higher than the affinity of WT NIS for I − ). Binding of NaB and the additional stabilization brought about by binding of multiple ions (Δg NaA,NaB , Δg NaA,ReO4 ) results in a triply occupied species that is only slightly less stable than the equivalent species in I − transport by WT NIS. In all three cases, the most stable species is the one that transitions to the inwardly facing conformation, ensuring that the most populated outwardly facing species is the one responsible for this crucial step of the transport cycle. In the absence of a transported anion, other populated species may sporadically transition and release their ion(s). This may account for the Na + currents observed in electrophysiological experiments carried out in the absence of an anion in Xenopus laevis oocytes expressing NIS [12] . The most remarkable property of NIS is probably its ability to transport I − , a very scarce ion, at the submicromolar concentrations prevailing in the extracellular milieu, given that it is difficult to bind a halide ion such as I − with high affinity [42] . Several aspects of the mechanism reported here provide insight into how NIS accomplishes this feat. Key to the process is the extracellular [Na + ]. Although the intrinsic affinity of NIS for I − is low ( K d,I =223 μM), it is 10 times higher ( K d,I 2 =22.4 μM) when Na + is already bound to the transporter. However, this K d is still one or two orders of magnitude higher than the concentrations of I − available under typical physiological conditions [43] , [44] , [45] . NIS overcomes this problem by taking advantage of the physiological [Na + ] and the increase in affinity for the second Na + (NaB) when the first Na + (NaA) site is occupied: at physiological [Na + ], ~79% of NIS molecules (calculated using the constants in Table 1 ; see also Fig. 3 and 6 ) are occupied by two Na + ions, and hence ready to bind and transport I − . That is, under physiological conditions, NIS is poised to bind and transport I − even when the [I − ] is well below its K d,I 2 . The fraction of NIS molecules that will transport I − depends on the extracellular [I − ]. Since the K d,I 2 for I − is ~22 μM, the fraction of transporting molecules at low [I − ] (that is, in the linear portion of the Michaelis–Menten versus [I − ] curve) will be ~79% of [I − ]/22 (both in μM), making NIS-mediated I − transport a remarkably efficient process. More to the point, at the physiological [Na + ], the fraction f of NIS molecules with I − bound that are triply occupied [ f =E 2Na,I /(E I +E Na,I +E 2Na,I )] remains essentially constant at a high value (87%) even when [I − ] changes from 1 to 0.1 or 0.01 μM. In other words, for a wide range of [I − ]s, close to 90% of NIS molecules with I − bound are in the form that can transition to the inwardly open conformation. 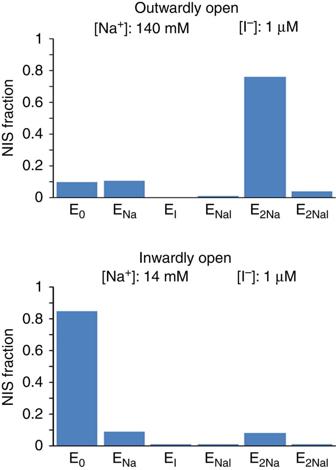Figure 6: Fraction of each of the ion bound species at typical ion concentrations in the extracellular milieu and the cytoplasm. The fractions under both sets of conditions were estimated using the constants inTable 1. The [I−] were arbitrarily set at 1 μM. At [Na+]=140 mM (outwardly open) the major species contains two bound Na+ions. At [Na+] =14 mM (inwardly open) empty NIS is the most abundant species. Figure 6: Fraction of each of the ion bound species at typical ion concentrations in the extracellular milieu and the cytoplasm. The fractions under both sets of conditions were estimated using the constants in Table 1 . The [I − ] were arbitrarily set at 1 μM. At [Na + ]=140 mM (outwardly open) the major species contains two bound Na + ions. At [Na + ] =14 mM (inwardly open) empty NIS is the most abundant species. Full size image Under conditions of severe I − scarcity, the rate of transport will likely be too low to overcome the rate of I − leakage and allow I − accumulation. Thus, without changing the mechanism, the only way to increase the transport rate and the resulting level of I − accumulation is to increase the number of NIS molecules. This may explain at the kinetic level why, under conditions of extreme I − scarcity, the long-term physiological response is to enlarge the thyroid gland (goitre) [46] . Completion of the transport cycle requires that all ions be released when the transporter is in the inwardly open conformation. One simple way to accomplish this would be for NIS to significantly reduce its affinity for the transported ions. Although this might occur, the ion affinities determined here for the different NIS species suggest a simpler mechanism in which the affinities of NIS for the transported ions are similar in the outwardly and the inwardly open conformations, analogously to what happens with other transporters [47] , [48] . [Na + ] inside the cell is typically 14 mM. If the affinity for the second Na + (NaB) in the inwardly facing conformation is similar to that in the outwardly facing conformation ( K d,NaB =19 mM), then a large percentage of NIS molecules (~70%) will lose both Na + ions; as a result, their affinity for I − will decrease and the anion will be released (~84% of NIS molecules will be empty and only 0.35% will have I − bound; Fig. 6 ). As the empty molecules switch to the outwardly facing conformation, a steady state will be established in which only a small percentage of inwardly facing molecules still have I − bound. As the ratio of outwardly to inwardly facing molecules is close to 1, most of the I − will be released into the cytoplasm. Interestingly, the fact that at the physiological [Na + ] most of the I − being transported binds NIS after two Na + ions have already bound seems to imply a Na + -Na + -I − binding order. However, this is not a mechanistic requirement: under non-physiological conditions, such as low Na + and high I − , one I − and one Na + will bind NIS in no particular order. The only mechanistic requirement is that binding of Na + to the second site (NaB) only takes place when the first Na + site (NaA) is already occupied. The insights offered here suggest that the binding properties of NIS maximize its ability to transport I − under physiological conditions. Given the environmental scarcity of this vital anion, NIS seems to be ‘making the most of a bad situation.’ The approach presented here provides an outstanding platform for studies of the effects of NIS mutations, including those found in patients with congenital iodide transport defects [49] . Moreover, it promises to be applicable to a wide variety of transporters, transport ATPases and channels. The ability to calculate the populations of species contributing to transport and their free energies from kinetic data obtained from whole cells, without having to purify and reconstitute the proteins, represents a significant advance towards elucidating the mechanism of these physiologically and medically relevant molecules. Cell culture The rat intestinal epithelial cell line IEC-6 was obtained from the American Type Culture Collection (Manassas, VA, USA). Cells were cultured in Dulbecco’s modified Eagle’s medium (Sigma-Aldrich) containing 4.5 g l −1 L -glucose, 3.7 g l −1 sodium bicarbonate, and 4 mM L -glutamine and supplemented with 0.1 U ml −1 bovine insulin and 10 % heat-inactivated fetal bovine serum (Gibco, Langley, OK, USA) [2] , [29] . Madin–Darby canine kidney cells stably expressing G93T hNIS were cultured as described [13] . Initial rates of I − and ReO 4 − transport To determine the initial rates of anion transport, 125 I − or 186 ReO 4 − was incubated for 2 min in the presence of the concentrations used, released with ice-cold ethanol, and quantified in a Cobra II Gamma Counter (Packard Bioscience, Meriden, CT, USA). For standardization, the amount of DNA per well was determined by the diphenylamine method after trichloroacetic acid precipitation [50] . Perrhenate kinetics ReO 4 − kinetic analyses were performed as described [13] , [20] . IEC-6 cells were incubated for 2 min with 0.075 to 100 μM 186 ReO 4 − (100 μCi μmol −1 ) (University of Missouri, Columbia, MO, USA) in the presence of no Na + or 17.5, 35, 70 or 140 mM Na + , keeping the osmolarity constant (140 mM) with choline chloride. Background, obtained with cells incubated in the absence of Na + , was subtracted. For Na + -dependent kinetic analysis of ReO 4 − transport, cells were incubated for 2 min with either 1.5, 3, 6 or 12 μM ReO 4 − (100 μCi μmol −1 ) at a range of Na + concentrations between 0 and 260 mM, keeping the osmolarity constant (260 mM) with choline chloride. Background obtained in cells at 0 mM Na + was subtracted from all points. All 232 points obtained in the four experiments (two varying [ReO 4 − ] at four different [Na + ]s and two varying [Na + ] at four [ReO 4 − ]s) were measured in triplicate. Fitting the initial rates data from individual experiments to the Michaelis–Menten equation with a Hill coefficient of 1.0 confirmed that NIS transports perrhenate with a 1:1 stoichiometry [20] . One example of such an adjustment varying [Na + ] (upper panel) and one varying [ReO 4 − ] (lower panel) are shown in Supplementary Fig. 2A . The apparent K M of Na + varies between 152.8 and 53.3 mM (upper panel), and that of ReO 4 − varies between 29.9 and 9.3 μM (lower panel). The apparent K M of each ion varies with the concentration of the other, suggesting that each one can bind to the free transporter and that each one influences the transporter’s affinity for the other. This was confirmed by fitting the experimental points to equation (5), which shows that binding of one ion increases the affinity of NIS for the other by a factor of 5.3 (Δ g Na,ReO4 ≈−1 kcal mol −1 ). In the panels of Supplementary Fig. 2b , the same experimental data used in Supplementary Fig. 2a are shown with curves obtained by substituting the parameters from Table 1 into equation (5). Remarkably, the quality of the global adjustment (panels b) is comparable to that obtained by fitting the individual curves (panels a), even though the data were fitted using only 4 parameters to fit the 232 experimental points, while adjustments of the individual experiments used 2 parameters to fit the data of each the 16 experiments (32 parameters total). Iodide kinetics I − kinetic analyses were performed as described [14] , [19] . IEC-6 cells were incubated for 2 min with 1.25 to 160 μM 125 I − (50 μCi μmol −1 ; Perkin-Elmer, Boston, MA, USA) in the presence of no Na + or 17.5, 35, 70 or 140 mM Na + , keeping the osmolarity constant (140 mM) with choline chloride. Background, obtained with cells incubated in the absence of Na + , was subtracted. For Na + -dependent kinetic analysis of I − transport, cells were incubated for 2 min with either 5, 10, 20 or 60 μM I − (50 μCi μmol −1 125 I − ) at a range of Na + concentrations between 0 and 260 mM, keeping the osmolarity constant (260 mM) with choline chloride. All 254 points obtained were measured in triplicate. Background, obtained in cells at 0 mM Na + , was subtracted. Michaelis–Menten analysis of the individual experiments using a Hill coefficient of 2 for Na + (ref. 12 ) shows that the apparent K M of each ion varies with the concentration of the other ( Supplementary Fig. 1A ), suggesting that each one can bind to the free transporter and that each one influences the transporter’s affinity for the other, in agreement with the results obtained using equation (3), which show that one Na + and one I − can bind to the empty transporter, and that binding of one of the ions enhances the transporter’s affinity for the other by a factor of 11.5 (Δ g Na,I ≈−1.5 kcal mol −1 ). Furthermore, when the same data used in Supplementary Fig. 1a were plotted using equation (3) and the parameters from Table 1 , the quality of the fit was virtually identical (panels b). This is remarkable given that only 5 parameters were used in the global fitting (the affinity for Na + was obtained from the ReO 4 − data), while 42 parameters (2 parameters for each experiment) would have been necessary to adjust the individual curves. More importantly, using equation (3) provides thermodynamic information about the interaction of the ions with the empty transporter (Δ G o NaA ≈−1.2 kcal mol −1 ; Δ G o I ≈−4.9 kcal mol −1 ) as well as the free energy of interaction (Δg Na,I ≈−1.5 kcal mol −1 ) and the affinity of the already occupied transporter for the second Na + (Δ G o NaA,NaB ≈−2.4 kcal mol −1 ). Statistical thermodynamics analysis The analysis follows the method of Shea and Ackers [23] using the nomenclature of Murphy and Freire [26] . The partition function is written using the Gibbs free energy of the eight macroscopic states ( Fig. 1 ) corresponding to the ion occupation of NIS. The empty transporter is taken as the ground state, and its Gibbs free energy is therefore set to zero. The Gibbs free energy of states E 1 , E 2 and E 3 in Fig. 1 ( G i ) is the Gibbs free energy of the state minus the free energy of the ground state ( , where [X] is the concentration of the free ion X). The Gibbs free energy of states E 4 , E 5 , E 6 and E 7 is expressed as a sum of two terms: (1) the sum of the Gibbs free energy of the states with a single ion for all ions in the state and (2) the free energy of interaction between all pairs of ions in that state (Δ g x,y ). The statistical weight of the different states is expressed as where is the product of the association constants ( ) of each individual ion to empty NIS,{ φ x,y } is the product of the enhancement in binding affinity experienced by ion x or y when the other ion is already bound ( ), and {[X x ]} is the product of the free concentrations of the ions bound in species i . The eight states and their statistical weights are shown in Supplementary Table 1 . How to cite this article: Nicola, J. P. et al . Physiological sodium concentrations enhance the iodide affinity of the Na + /I − symporter. Nat. Commun. 5:3948 doi: 10.1038/ncomms4948 (2014).